Giraffe genome sequence reveals clues to its unique morphology and physiology The origins of giraffe’s imposing stature and associated cardiovascular adaptations are unknown. Okapi, which lacks these unique features, is giraffe’s closest relative and provides a useful comparison, to identify genetic variation underlying giraffe’s long neck and cardiovascular system. The genomes of giraffe and okapi were sequenced, and through comparative analyses genes and pathways were identified that exhibit unique genetic changes and likely contribute to giraffe’s unique features. Some of these genes are in the HOX, NOTCH and FGF signalling pathways, which regulate both skeletal and cardiovascular development, suggesting that giraffe’s stature and cardiovascular adaptations evolved in parallel through changes in a small number of genes. Mitochondrial metabolism and volatile fatty acids transport genes are also evolutionarily diverged in giraffe and may be related to its unusual diet that includes toxic plants. Unexpectedly, substantial evolutionary changes have occurred in giraffe and okapi in double-strand break repair and centrosome functions. The origin of giraffe’s iconic long neck and legs, which combine to elevate its stature to the tallest terrestrial animal, has intrigued mankind throughout recorded history and became a focal point of conflicting evolutionary theories proposed by Lamarck and Darwin. Giraffe’s unique anatomy imposes considerable existential challenges and three systems bear the greatest burden: the cardiovascular system to maintain blood pressure homeostasis [1] , the musculoskeletal system to support a vertically elongated body mass [2] and the nervous system to rapidly relay signalling over long neural networks [3] , [4] . To pump blood vertically 2 m from the heart to the brain giraffe has evolved a turbocharged heart and twofold greater blood pressure than other mammals [1] , [5] . The blood vessel walls in the lower extremities are greatly thickened to withstand the increased hydrostatic pressure, and the venous and arterial systems are uniquely adapted to dampen the potentially catastrophic changes in blood pressure when giraffe quickly lowers its head to drink water [1] , [5] , [6] , [7] , [8] , [9] , [10] , [11] . To sustain the weight of the long neck and head, the nuchal ligament, which runs down the dorsal surface of the cervical vertebrae and attaches to the anterior thoracic vertebrae, is greatly enlarged and strengthened [2] , [12] . Okapi ( Okapia johnstoni ), the giraffe’s closest relative and the only other extant member of the Giraffidae family, provides a useful comparison, because it does not share these unique attributes seen in giraffe [13] . Nine subspecies of giraffe have been identified that can be distinguished by coat colour and pattern, and have been reproductively isolated as long as 2 mya (refs 14 , 15 ). Two giraffe subspecies are nearly extinct and overall the number of giraffes have declined by 40% since 2000, due to poaching and habitat loss [16] . As all giraffe subspecies share the unique anatomical and physiological adaptation of the giraffe genus, they provide an important cross-check for unique patterns of genetic variation. Here we sequenced the genomes of the Masai giraffe and okapi, and through comparative analysis with other eutherians mammals, 70 genes were identified that exhibit multiple signs of adaptation (MSA) in giraffe. Several of these genes encode well-known regulators of skeletal, cardiovascular and neural development, and are likely to contribute to giraffe’s unique characteristics. Genome sequencing and de novo assembly The whole-genome sequence of two Masai giraffe ( Giraffa camelopardalis. tippelskirchi ) from the Masai Mara (MA1) in Kenya and the Nashville Zoo (NZOO), and one fetal okapi ( O. johnstoni ) from the White Oak Conservatory was determined by constructing paired-end libraries followed by sequencing using an Illumina HiSeq yielding ca . 30 × coverage. Mate-paired libraries were also prepared from the MA1 Masai giraffe and okapi, and sequenced to increase coverage and to span repetitive sequence elements. 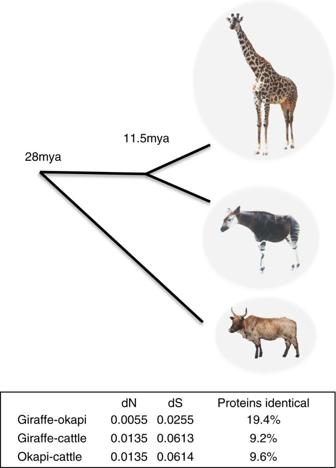Figure 1: Divergence of giraffe and okapi from a common ancestor. Using the average pairwise synonymous substitution divergence (dS) estimates between giraffe, okapi and cattle as calibrated by the pecoran common ancestor (27.6 mya), the divergence of giraffe and okapi from a common ancestor is estimated to be 11.5 mya. Okapi image adapted from a photograph by Raul654. The initial sequence reads from giraffe and okapi were aligned to the 19,030 cattle (Bos taurus) references transcripts [17] to predict homologous genes ( Supplementary Table 1 ), which yielded 17,210 giraffe and 17,048 okapi genes. 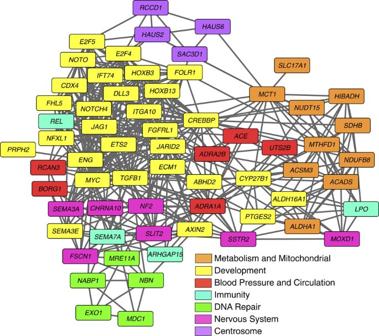Figure 2: Network analysis of GO biological process of giraffe MSA genes. Seventy genes were identified that exhibited MSAs based on amino acid sequence divergence as evaluated by neighbour-joining phylogenetic analysis of mammalian orthologous proteins, enrichment of nonsynonymous substitutions, unique amino acid substitutions at sites otherwise fixed in mammals, substitutions predicted to cause functional changes by Polyphen2 analysis and substitutions under positive selection. Cluster analysis was performed on the set of 70 giraffe MSA genes based on GO Biological Process using Cytoscape 3.0 (ref.68). The giraffe and okapi sequence data were also used to generate a draft genome assembly with a total length of 2.9 and 3.3 Gb for giraffe and okapi, respectively ( Supplementary Table 2 ). To verify gene predictions and gene structure in cases where the original gene annotations for giraffe and okapi were incomplete or ambiguous, the draft assembly was aligned to dog or human gene sequences. To determine whether substitutions unique to Masai giraffe were conserved in other giraffe subspecies, we performed targeted sequencing of several genes in Rothschild ( G.c. rothschildi ) and Reticulated ( G.c. reticulata ) giraffes, which diverged from Masai giraffe ∼ 1-2 mya (refs 15 , 18 ). Comparative genome analysis To identify changes that potentially underlie these unique morphological and physiological adaptations, we analysed the coding sequences of orthologous genes in giraffe, okapi and cattle. Giraffe and okapi genes are highly similar overall with 19.4% of proteins being identical ( Fig. 1 ). Giraffe and okapi genes are equally distantly related to cattle, suggesting that giraffe’s unique characteristics are not due to an overall faster rate of evolution. The divergence of giraffe and okapi, based on the relative rates of synonymous substitutions, from a common ancestor is estimated to be 11.5 mya ( Fig. 1 ), substantially less than the previous estimate of 16 mya (refs 19 , 20 ), which was based on mitochondrial DNA sequence comparisons. Figure 1: Divergence of giraffe and okapi from a common ancestor. Using the average pairwise synonymous substitution divergence (dS) estimates between giraffe, okapi and cattle as calibrated by the pecoran common ancestor (27.6 mya), the divergence of giraffe and okapi from a common ancestor is estimated to be 11.5 mya. Okapi image adapted from a photograph by Raul654. Full size image Adaptive evolution of giraffe Adaptive divergence was evaluated by pairwise analysis of 13,581 giraffe, okapi and cattle genes that showed at least 90% coverage by comparing nonsynonymous (dN) changes in protein coding sequences as well as normalized to synonymous (dS) changes (dN/dS, ω ). Enrichment analysis based on gene function (gene ontology (GO) biological processes) and pathway relationships Kyoto Encyclopedia of Genes and Genomes (KEGG) revealed elevation of dN or ω for giraffe in genes related to metabolism (tricarboxylic acid cycle, oxidative phosphorylation and butyrate), growth and development (cell proliferation, skeletal development and differentiation), the nervous system and cardiac muscle contraction ( Supplementary Table 2 ). In parallel, we employed Polyphen2 analysis [21] to identify genes that contain amino acid substitutions that are predicted to cause a significant alteration in function and screened for genes that exhibited evidence for positive selection. 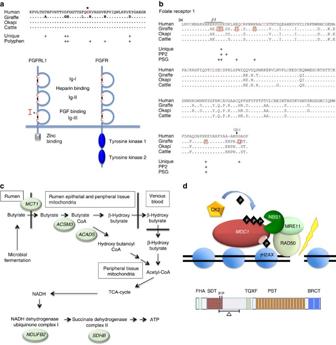Figure 3: Giraffe genes and pathways exhibiting extraordinary divergence and patterns of amino acid substitutions. (a) GiraffeFGFRL1contains seven amino acid substitutions that are unique at fixed sites in other mammals and/or are predicted by Polphen2 analysis to alter function (upper panel). Human reference is shown, which is identical to cattle and okapi in this segment. The unique giraffe substitutions occur in the FGF-binding domain region flanking the N-terminal cysteine (asterisk) of the Ig-III loop (lower panel). Red bracket in lower panel corresponds to the sequence in the upper panel. The extracellular structure of FGFRL1 (left) is the same as a prototypical FGF receptor (FGFR, right) but lacks the cytoplasmic C-terminal tyrosine kinase domains seen in FGFR and instead contains a zinc-binding domain. (b) GiraffeFOLR1contains seven substitutions that each show evidence of positive selection (P<0.05) by the branch-site model. Two of the positive selected sites (PSG), P48S and E222K, are also unique substitutions at fixed sites and Polyphen2 (PP2) analysis predicts them to alter function. P48S is withinβ-sheet-1 that forms part of the folic acid-binding pocket. The FOLR1 protein forms a globular structure maintained by overlapping disulfide bridges between 16 cysteine residues (red) and tethered to the plasma membrane at S233 by a Gpi anchor. The unique substitution in giraffe, G234Q, immediately adjacent to the Gpi anchor site may alter the anchor site or the rate of its formation. (c) Genes encoding key enzymes in butyrate metabolism and downstream mitochondrial oxidative phosphorylation pathways have diverged in giraffe including the monocarboxylate transporter (MCT1), acyl-coenzyme A synthetase-3 (ACSM3), short-chain specific acyl-CoA dehydrogenase (ACADS), NADH dehydrogenase (ubiquinone) 1β subcomplex subunit 2 (NDUFB2) and succinate dehydrogenase [ubiquinone] iron-sulfur subunit (SDHB).ACSM3andACADSare located in the mitochondrial matrix where asNDUFA2,NDUFB2andSDHBare located in the mitochondrial inner membrane. In addition to being present in the rumen epithelial cells, MCT1 is highly expressed in the heart, skeletal muscle and the nervous system where it acts to transport volatile fatty acids (VFAs) and lactate. (d) Double-strand break repair genes exhibit divergence in giraffe and/or okapi. The mediator of DNA-damage check point 1 (MDC1) binds phosphorylated H2AX, which mark DNA double-strand break, and serves as scaffold to recruit the MRN DNA repair complex composed of NBS1, MRE11 and RAD50 (upper panel). The giraffe and okapiMDC1gene exhibits a 264 amino acid deletion that removes part of the SDT region that harbours two critical CK2 phosphorylation sites (lower panel). These two phosphorylation sites are among multiple sites that regulate the interaction of MDC1 and NBS1 essential for the recruitment of the MRN complex to double-strand breaks. Genes exhibiting positive selection in giraffe were enriched in lysosomal transport, natural killer cell activation, immune response, angiogenesis, protein ADP ribosylation, blood circulation and response to pheromones ( Supplementary Table 3 ). Over 400 genes were identified from the giraffe–okapi–cattle analysis that exhibited some degree of genetic differentiation in giraffe by the aforementioned analysis. These selected genes were further compared with orthologues across a large set of mammals, including 14 other cetartiodactyls, to more fully assess evidence of positive selection, relative amino acid sequence divergence and to identify amino acid substitutions unique to giraffe among eutherians. 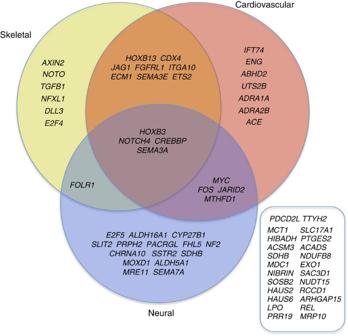Figure 4: Gene cluster analysis of genes that exhibit evidence of adaptive evolution in giraffe. Developmental and physiological regulatory genes in giraffe that exhibit adaptive evolution are enriched in skeletal, cardiovascular and neural functions. The MSA genes that are not known to be related to the regulation of skeletal, cardiovascular, or neural development are listed (right box). Seventy genes displayed MSA in giraffe by these criteria ( Supplementary Table 4 and Supplementary Fig. 1 ). The unique amino acid substitutions identified in these genes were confirmed in the two unrelated individual Masai giraffe and, in some cases, confirmed in Reticulated and Rothschild giraffe by targeted sequencing. Network analyses based on GO biological process revealed eight functional clusters among the 70 MSA genes including development, cell proliferation, metabolism, blood pressure and circulation, nervous system, double-strand DNA break repair, immunity and centrosome function ( Fig. 2 ). Remarkably, nearly half of these genes are involved in controlling developmental pattern formation and differentiation including homeobox, Notch, Wnt and fibroblast growth factor (FGF) pathway genes, major regulators of growth and cell proliferation including the transcription factors MYC, E2F4, E2F5, ETS2, TGFB1 and CREBBP, and the folate receptor 1 (FOLR1). Figure 2: Network analysis of GO biological process of giraffe MSA genes. Seventy genes were identified that exhibited MSAs based on amino acid sequence divergence as evaluated by neighbour-joining phylogenetic analysis of mammalian orthologous proteins, enrichment of nonsynonymous substitutions, unique amino acid substitutions at sites otherwise fixed in mammals, substitutions predicted to cause functional changes by Polyphen2 analysis and substitutions under positive selection. Cluster analysis was performed on the set of 70 giraffe MSA genes based on GO Biological Process using Cytoscape 3.0 (ref. 68 ). Full size image Evolution of regulators of skeletal growth and differentiation The extraordinarily long neck of giraffe is not due to adding cervical vertebrae as is the case for long-necked birds, but rather to the vertical extension of each of the seven prototypical cervical vertebrae present in mammals [13] , [22] . The elongation of the cervical vertebrae in giraffe is probably due to the extension of somites, which give rise to the cervical vertebrae during early embryogenesis [22] , and is restricted to the cervical region by the combinatorial action of homeobox genes. The major genes and developmental pathways that specify vertebrae differentiation of the axial and appendicular skeleton in giraffe and okapi were compared with other mammals to determine whether unique patterns of amino acid substitutions were found in giraffe ( Supplementary Table 5 ). The homeobox genes HOXB3 , CDX4 and NOTO exhibit enhanced divergence in giraffe among eutherians and have unique amino acid substitutions predicted to alter protein function. In addition, HOXB13 , which regulates angiogenic and posterior axial skeletal development, shows high amino acid sequence divergence in giraffe and okapi compared with other mammals ( Supplementary Table 4 ). Modulating the posterior to anterior gradient of fibroblast growth factor signalling or changing the cyclical expression of genes in the NOTCH or WNT signalling pathways could potentially modulate somite size. We found that FGFRL1 , a decoy FGF receptor, AXIN2 , a negative regulator of the WNT pathway, and three genes in the NOTCH pathway including NOTCH4 , JAG1 and DLL3 exhibit amino acid sequence divergence in giraffe and exhibited multiple unique amino acid substitutions compared with other eutherians. The divergence of giraffe FGFRL1 is particularly striking with a cluster of seven unique substitutions ( Fig. 3a ) in the domain that interacts with FGF ligands. FGFRL1 is among nine genes in giraffe that exhibit a significantly higher number of unique amino substitutions at fixed sites in mammals ( Supplementary Table 4 ). FGFRL1 in mammals lacks a tyrosine kinase domain essential for downstream FGF signalling and acts as a competitive inhibitor of the nascent FGF receptors [23] . Interestingly, Badlangana et al . [22] speculated that an inhibitor of FGF signalling might be responsible for modulating the size of giraffe cervical vertebrae based on the discovery that chemical inhibition of FGF signalling increased somite size in the chick embryo [24] . Consistent with its hypothesized role in regulating unique features of giraffe, FGFRL1 mutations in mice and human display severe defects in skeletal and cardiovascular development [25] , [26] , [27] . Figure 3: Giraffe genes and pathways exhibiting extraordinary divergence and patterns of amino acid substitutions. ( a ) Giraffe FGFRL1 contains seven amino acid substitutions that are unique at fixed sites in other mammals and/or are predicted by Polphen2 analysis to alter function (upper panel). Human reference is shown, which is identical to cattle and okapi in this segment. The unique giraffe substitutions occur in the FGF-binding domain region flanking the N-terminal cysteine (asterisk) of the Ig-III loop (lower panel). Red bracket in lower panel corresponds to the sequence in the upper panel. The extracellular structure of FGFRL1 (left) is the same as a prototypical FGF receptor (FGFR, right) but lacks the cytoplasmic C-terminal tyrosine kinase domains seen in FGFR and instead contains a zinc-binding domain. ( b ) Giraffe FOLR1 contains seven substitutions that each show evidence of positive selection ( P <0.05) by the branch-site model. Two of the positive selected sites (PSG), P48S and E222K, are also unique substitutions at fixed sites and Polyphen2 (PP2) analysis predicts them to alter function. P48S is within β -sheet-1 that forms part of the folic acid-binding pocket. The FOLR1 protein forms a globular structure maintained by overlapping disulfide bridges between 16 cysteine residues (red) and tethered to the plasma membrane at S233 by a Gpi anchor. The unique substitution in giraffe, G234Q, immediately adjacent to the Gpi anchor site may alter the anchor site or the rate of its formation. ( c ) Genes encoding key enzymes in butyrate metabolism and downstream mitochondrial oxidative phosphorylation pathways have diverged in giraffe including the monocarboxylate transporter ( MCT1 ), acyl-coenzyme A synthetase-3 ( ACSM3 ), short-chain specific acyl-CoA dehydrogenase ( ACADS ), NADH dehydrogenase (ubiquinone) 1β subcomplex subunit 2 ( NDUFB2 ) and succinate dehydrogenase [ubiquinone] iron-sulfur subunit ( SDHB ). ACSM3 and ACADS are located in the mitochondrial matrix where as NDUFA2 , NDUFB2 and SDHB are located in the mitochondrial inner membrane. In addition to being present in the rumen epithelial cells, MCT1 is highly expressed in the heart, skeletal muscle and the nervous system where it acts to transport volatile fatty acids (VFAs) and lactate. ( d ) Double-strand break repair genes exhibit divergence in giraffe and/or okapi. The mediator of DNA-damage check point 1 (MDC1) binds phosphorylated H2AX, which mark DNA double-strand break, and serves as scaffold to recruit the MRN DNA repair complex composed of NBS1, MRE11 and RAD50 (upper panel). The giraffe and okapi MDC1 gene exhibits a 264 amino acid deletion that removes part of the SDT region that harbours two critical CK2 phosphorylation sites (lower panel). These two phosphorylation sites are among multiple sites that regulate the interaction of MDC1 and NBS1 essential for the recruitment of the MRN complex to double-strand breaks. Full size image The Giraffe FOLR1 shows exceptionally strong evidence for adaptive evolution including six positively selected amino acid substitutions of which two are predicted to cause a significant change in function ( Fig. 3b ). FOLR1 mutations are embryonically lethal in mice [28] and produce hypomyelination and neurological defects in humans [29] . In addition to its role in cellular folate transport, FOLR1 is internalized, processed and transported to the nucleus where it regulates components of the FGF and NOTCH pathways [30] . These changes in giraffe FOLR1 may act in concert with similar changes in FGFRL1 and JAG1 , components of the FGF and NOTCH pathways, respectively, to forge major developmental adaptations. Cardiovascular and metabolic gene evolution The giraffe cardiovascular system is adapted to regulate blood pressure over a height of 6 m and to maintain cardiovascular homeostasis associated with rapid changes in the relative position of the brain to the heart. The blood pressure of giraffe is 2.5 × higher than man, the left ventricle of the heart is enlarged and the blood vessel walls of the lower extremities are greatly thickened [1] , [31] . Giraffe exhibits evidence for adaptive evolution of eight genes that regulate blood pressure or cardiovascular function including two of the major adrenergic receptors α1 and β-2, urotensin-2b and angiotensin-converting enzyme ( Supplementary Table 4 ). BORG1 and RCAN3, which are highly expressed in the heart and purported to have important functions related to cell shape and cardiac muscle contraction, respectively, are also significantly diverged in giraffe [32] , [33] . The observed distinctive changes in these genes may provide clues as to the evolutionary origins of giraffe’s high blood pressure, increased cardiac output and modified vasculature. Giraffe’s elevated stature enables it to feed on acacia leaves and seedpods that are highly nutritious but also contain toxic alkaloids. As with other ruminants, giraffes’ gut microbes ferment plants to generate volatile fatty acids that are transported through the gut epithelium and serve as the main energy source [34] , [35] . Included among the MSA genes in giraffe are those involved in the catabolism of volatile fatty acids such as butyrate (MCT1, ACSM3 and ACADS) or downstream oxidative phosphorylation that generate ATP (NDUB2 and SDHB) ( Fig. 3c ). In addition, these proteins are essential for lactate transport and metabolism that is particularly important for cardiovascular functions [36] . Evolutionary changes in DNA and chromosome repair genes The mediator of damage checkpoint-1 (MDC1) acts as a key scaffold for proteins participating in double-strand DNA break repair, homologous recombination, nonhomologous end-joining and telomere maintenance [37] , [38] , [39] , [40] , [41] , [42] , [43] , and its sequence exhibits the most radical evolutionary change in giraffe and okapi compared with all other vertebrates. The giraffe and okapi MDC1 gene contains an in-frame termination substitution in exon 5, suggesting either premature termination or alternative splicing to remove the offending termination codons. The complementary DNAs from both giraffe and okapi liver tissue were truncated in exon 5, indicating the use of a cryptic 5′-splice site resulting in a 264-amino acid internal deletion not seen in any other vertebrate. The deleted region corresponds to the ST/Q domain that contains numerous phosphorylation sites that have an impact on important regulatory protein–protein interactions [44] . Perhaps, not surprisingly, the amino acid sequence of NIBRIN, MRE11 and SOSB2, and BAZB1, which interact with MDC1 (ref. 45 ) are diverged in giraffe and/or okapi ( Fig. 3d ). We speculate that the divergence of these genes and those involved in centromeric functions may underlie the unusual degree of chromosomal fusions that occurred in the giraffe lineage [46] , [47] . The pecoran ancestor that gave rise to the horned, even-toed ungulates is purported to have had a karyotype of 2 n =58–60 as exemplified by cattle [46] . However, giraffe and okapi have unusual karyotypes among pecorans exhibiting reduced chromosome number of 2 n =30 and 2 n =44–46, respectively, due to Robertsonian centric fusions of acrocentric chromosomes. Genes regulating fundamental aspects of development and physiology are highly conserved among major mammalian taxa [48] , [49] . However, we found that two-thirds of the genes most diverged in giraffe have specific roles in regulating skeletal, cardiovascular and/or neural development, or physiology ( Fig. 4 ). In addition, several identified genes functionally intersect metabolism, growth and cardiovascular function, suggesting that giraffe’s unique features may have co-evolved to elevate its stature, adapt its metabolism for more toxic food sources and adapt its cardiovascular and nervous system to the increased demands imposed by its unique morphology. The camel’s neck is relatively long among mammals and intermediate in length between giraffe and okapi [22] . However, unlike the giraffe, the camel’s long neck does not function to increase its stature and we did not detect similar patterns of unique amino acid substitutions between giraffe and camel among the 70 giraffe MSA genes including those that are known to regulate skeletal development. Okapi shares some of the same genetic changes seen in giraffe, which for some genes might underlie shared adaptive traits, whereas in other cases might represent evolutionary remnants of a common Giraffidae ancestor that is purported to have had a shorter neck than giraffe but longer than that of okapi [50] . Figure 4: Gene cluster analysis of genes that exhibit evidence of adaptive evolution in giraffe. Developmental and physiological regulatory genes in giraffe that exhibit adaptive evolution are enriched in skeletal, cardiovascular and neural functions. The MSA genes that are not known to be related to the regulation of skeletal, cardiovascular, or neural development are listed (right box). Full size image Among the 70 genes exhibiting MSA in giraffe, FGFRL1 is the strongest candidate for directly having an impact on the unique growth of the axial and appendicular skeleton and the cardiovascular system. FGFRL1 is known to be essential for normal skeletal and cardiovascular development in humans and mice [25] , [26] , [27] , and the FGF pathway regulates somite size [51] . Other genes are required to restrict differential growth to the cervical vertebrae and legs, and the homeotic genes, which specify the identity of different regions of the body, probably play that role. We identified three homeobox genes— HOXB3 , CDX4 and NOTO —which exhibit significant changes in giraffe compared with other mammals. The advent of gene-editing methods provide a means of testing these hypotheses by introducing the unique amino acid substitutions seen in giraffe into the homologous genes of model organisms and determining the functional consequences. Among mammals, giraffe has some of the most challenging physiological and structural problems imposed by its towering height. The solutions to these challenges, in particular related to its turbocharged circulatory system, may be instructive for treatment of cardiovascular disease and hypertension in humans. Genome sequencing The Illumina TruSeq DNA PCR-Free Library Preparation Kit was used to construct paired-end libraries from liver samples of two female Masai giraffe ( G.c. tippelskirchi ) from the MA1 in Kenya and the Nashville Zoo (NZOO), and one fetal male okapi ( O. johnstoni ) from the White Oak Holdings. Libraries were prepared according to the manufacturer’s protocol using 2 μg of input and the 550 bp insert size workflow. The Nextera Mate Pair Sample Preparation Kit was used to construct mate pair libraries from the same three samples using the manufacturer’s ‘Gel Plus’ protocol with 4–8 kb size selection. Libraries were sequenced on an Illumina HiSeq 2500 in Rapid Run mode using 2 × 150-bp paired-end sequencing. All libraries were prepared and sequenced by the Penn State Genomics Core Facility at University Park, PA. Targeted sequencing of specific genes in Rothschild ( G.c. rothschildi) and Reticulated ( G.c. retulata) giraffe used genomic DNA that we isolated from primary fibroblast cell cultures obtained from Dr Oliver Ryder at the San Diego Zoo Institute for Conservation Research. Quality control and genome coverage Interspecies variant nucleotides were identified as follows. The sequences that aligned to the reference genome as described above were sorted by the start position of their alignment to the reference genome. These were then assembled using a reference-based approach [52] , requiring at least 2-fold and at most 80-fold coverage of the region to be considered for assembly. The sequences from the okapi samples were aligned to the giraffe consensus sequence using BWA [53] version 0.5.9 with default arguments and differences between giraffe and okapi were then identified using SAMtools [54] version 0.1.19 with default arguments and the mpileup command. In-house scripts (available on request) were used to determine the position of variants relative to the (cow or dog) reference sequence. Reads were discarded if the above process revealed evidence of insufficient read quality or instability of the genomic region, using three criteria. First, reads were required to have a best alignment to the reference assembly with at least 3% more identical nucleotides than the second-best alignment. Second, reference contigs were ignored if the depth of coverage was too high or too low according to the Lander–Waterman statistic. Third, regions with an unusually high putative rate of interspecies differences were ignored, to lessen the impact of duplications and low-complexity regions. The average depth of read coverage for the nucleotide differences identified using the dog reference assembly and applied in subsequent analyses were 20.0 for the giraffe from MA1, 21.6 for the Nashville Zoo (NZOO) giraffe and 16.8 for the okapi. Approximately 300 genes that displayed relative high dN/dS ratios in giraffe compared with cow and okapi were lacking complete coverage relative to cattle or other orthologues of other mammals. In most cases, incomplete coverage of these genes was due to the fact that the reference cattle gene model that was used was incomplete relative to other mammals. To complete the annotation for these genes, the giraffe and okapi scaffolds containing these genes were identified. The appropriate scaffolds were analysed by the Genewise [55] annotation programme using complete reference coding sequences from cattle or human. Ensembl reference transcripts with the highest degree of confidence and information (TSL:1, GENECODE basic, APPRIS P1) were used. De novo assembly First, TruSeq adapters from mate-pair data were removed using Nesoni default parameters (v0.115) ( https://github.com/Victorian-Bioinformatics-Consortium/nesoni ). Then, KmerGenie (v1.6269) [56] was executed with default parameters on both data sets, to determine best k-mer sizes for assembly. Scaffolds were assembled using SOAPdenovo2 (v2.04) [57] , setting k-mer size to 91 for the giraffe data set and 81 for the okapi data set, and enabling repeat resolution (-R parameter). Finally, gaps in scaffolds were filled using GapCloser (v1.12) with default parameters. The same paired-end and mate-pair reads that were used to assemble were mapped back to the giraffe and okapi assemblies. The BWA-MEM programme was executed with default parameters and statistics were extracted using the ‘samtools stats’ tool. It is noteworthy that the percentage of properly mapping mate pairs was lower than for paired ends, as the larger span of a mate pair makes it more likely to map across different scaffolds. Alignments and gene trees Before aligning sequences, tblastn was run on each sequence against corresponding cow protein RefSeq sequence (downloaded from Ensembl). This ensured correction for frame shifts indels, as it was noted that some sequences were of draft quality and may have some sequencing errors. Sequences were aligned using MUSCLE release 3.8 (ref. 58 ) and phylogenetic trees were constructed using PhyML Version 3.0 (ref. 59 ). PhyML uses a likelihood-based tree-searching algorithm to find an optimal phylogeny. Bootstrapping ( n =100) was used to test the robustness of the resulting phylogenies. Positive selection analyses To test for signatures of positive selection acting on giraffe lineage for each of the genes, we compared the likelihood scores of selection models implemented in CODEML in the PAML package, version 4.7 (ref. 60 ), using likelihood ratio tests (LRTs). Branch-site models were used to identify positive selection acting on giraffe versus cattle, okapi and gerenuk. The revised branch-site model A was used, which attempts to detect positive selection acting on a few sites on particular specified lineages, that is, ‘foreground branches’ [61] . Four classes of sites are assumed in the model and codons are categorized into these site classes based on foreground and background estimates of ω. The alternative hypothesis that positive selection occurs on the foreground branches (ω>1) is compared with the null hypothesis, where ω=1 is fixed, using an LRT [62] . All genes whose LRT χ 2 - analysis yielded P -values<0.05 were considered significant and these were selected as initial positive selection gene (PSG) candidates. As maximum likelihood methods designed to detect episodes of positive selection are sensitive to taxa sample size [63] , we re-analysed the initial PSG candidates list by including the orthologues of all mammals for which high-quality sequence data were available (10–45 species). In addition, genes identified by other means to have shown evidence of selection/divergence in giraffe were subjected to PSG analyses using all the available high-sequence quality mammalian orthologues. The results of the PSG analysis are given for the 70 MSA genes in Supplementary Table 4 . Bayesian empirical Bayes values [64] were used to identify sites under significant positive selection. Functional classification of positively selected genes was achieved using PANTHER classification of Biological Process ontology terms [65] . Evaluation of nucleotide and amino acid substitutions The mappings between giraffe–okapi nucleotide difference and the reference assembly allowed us to predict amino-acid difference (in the case of nonsynonymous protein-coding differences) as follows. Ensembl gene annotations identified protein-coding regions in the reference assembly, which were inferred to map to coding regions in giraffe and okapi, as well as revealing the transcription orientation and phase. These data were analysed extensively on the Galaxy platform [66] , [67] to determine enrichment of dN and dN/dS ( ω ) in giraffe–cattle as compared with okapi–cattle. Genes that exhibit higher dN or dN/dS values in the giraffe–cattle dyad were subjected to (a) KEGG pathway analysis and biological function analysis. Approximately 400 genes exhibiting exceptionally higher dN or dN/dS values in giraffe–cattle dyad were further analysed in detail including (a) Polyphen2 analysis [21] to identify amino acid substitutions predicted to be ‘probably damaging’; (b) Unique Substitution Analysis to identify unique amino acid substitutions in giraffe at fixed sites in eutherians, and to determine which genes have a statistically significant excess of unique substitutions at fixed sites, unique substitutions were manually curated from BLAST alignments; and (c) protein phylogenetic tree analysis using neighbour-joining method to identify genes that exhibit a high degree of divergence in giraffe as assessed by relative branch lengths. In assessing unique substitutions and constructing phylogenetic trees, all available mammalian orthologues of sufficient sequence quality were used. These data were combined with global analysis of positive selection analysis to identify genes that exhibit MSA in giraffe. This aggregate analysis led to the identification of 70 MSA genes. For these 70 genes, the amino acid substitutions unique to giraffe were confirmed in 2 individual Masai giraffes (MA1 and NZOO) and confirmed in an individual Rothschild and Reticulated giraffe including FGFRL1 , FOLR1 , RCAN3 , AXIN2 and HOXD9 . Accession codes: Sequence data for G. camelopardalis tippelskirchi (MA1 and NZOO) and O. johnstoni (WOAK) have been deposited in Short Read Archive under project number SRP071593 (BioProject PRJNA313910 ) and accession codes NZOO: SRX1624609 and MA1: SRX1624612. The Whole Genome Shotgun project of G. camelopardalis tippelskirchi (MA1) has been deposited at DDBJ/ENA/GenBank under the accession LVKQ00000000 and the version described in this paper is version LVCL01000000 . The Whole Genome Shotgun project of O. johnstoni (WOAK) has been deposited at DDBJ/ENA/GenBank under the accession LVCL00000000 and the version described in this paper is version LVCL01000000 . How to cite this article: Agaba, M. et al . Giraffe genome sequence reveals clues to its unique morphology and physiology. Nat. Commun. 7:11519 doi: 10.1038/ncomms11519 (2016).